A nanomechanical interface to rapid single-molecule interactions Single-molecule techniques provide opportunities for molecularly precise imaging, manipulation, assembly and biophysical studies. Owing to the kinetics of bond rupture processes, rapid single-molecule measurements can reveal novel bond rupture mechanisms, probe single-molecule events with short lifetimes and enhance the interaction forces supplied by single molecules. Rapid measurements will also increase throughput necessary for technological use of single-molecule techniques. Here we report a nanomechanical sensor that allows single-molecule force spectroscopy on the previously unexplored microsecond timescale. We probed bond lifetimes around 5 μs and observed significant enhancements in molecular interaction forces. Our loading-rate-dependent measurements provide experimental evidence for an additional energy barrier in the biotin–streptavidin complex. We also demonstrate quantitative mapping of rapid single-molecule interactions with high spatial resolution. This nanomechanical interface may allow studies of molecular processes with short lifetimes and development of novel biological imaging, single-molecule manipulation and assembly technologies. Precise recognition mechanisms of biological molecules offer a tremendous potential for the assembly [1] , [2] , [3] , imaging [4] , [5] and analysis of complex biological materials [6] . Single-molecule force spectroscopy (SMFS) experiments with the atomic force microscope (AFM) [7] have demonstrated the potential of intermolecular forces to be used for chemically specific nanoscale imaging [8] , manipulation [9] , directed assembly [10] , and biophysical studies of deformation and failure of biomolecules [11] . Forces measured during the rupture of molecular bonds are affected by thermally activated dissociation, which results in loading-rate-dependent characteristics. Consequently, the slow mechanical interface to single-molecule processes makes it difficult to access short-lived single-molecule events [12] . For example, a comparison of experiments and molecular dynamics (MD) simulations of the well-studied biotin–avidin complex shows that these molecules have a potential to supply forces much larger than that encountered in experiments [13] , [14] , [15] . The larger forces will emerge only if bound molecules are pulled apart on a shorter timescale. Furthermore, experimental access to short timescales can provide insights into failure of protein-based materials in which failure mechanisms depend on the timescales of external forces [16] . In principle, SMFS can be integrated into the tapping-mode imaging platform, where the cantilever oscillates back and forth against the surface on resonance and at a high frequency. Evidence for this is provided by the molecular recognition images obtained in the topography and recognition imaging mode (TREC) [5] . In this mode, molecular binding events produce detectable patterns in the oscillation amplitude. This suggests that single molecules can efficiently bind and unbind at the short timescales offered by the resonating microcantilever. If a rapid nanomechanical interface to these interactions is built, high-speed SMFS can be obtained at the frequency of the vibrating cantilever. In this study, we have designed an AFM cantilever that establishes a rapid nanomechanical interface to single-molecular interactions, thereby increasing the rate of SMFS by nearly four orders of magnitude. The new design is using the torsional harmonic cantilever concept that was developed for high-resolution nanomechanical analysis of samples [17] , [18] . These T-shaped cantilevers generate high-speed force-distance curves during the tapping-mode AFM imaging process. Measurements carried out with this nanomechanical interface allowed explorations of single-molecule processes on the microsecond timescale. Analysis of the rupture forces of the well-studied biotin–streptavidin complex at the short timescales has provided experimental evidence for an additional energy barrier. The high speed of measurements further allowed generating high-resolution maps of the quantitative rupture forces. 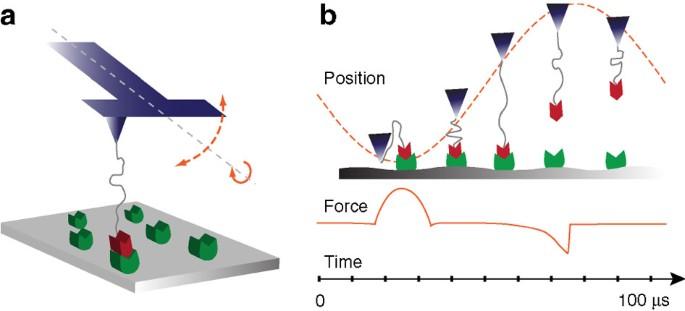Figure 1: Schematic of SMFS on the microsecond timescale. (a) The ligand is attached to a specially designed T-shaped AFM cantilever via a flexible polymer spacer. Tip-sample interactions twist the vibrating cantilever. The vertical deflection signal gives the tip position, and the twist angle gives the instantaneous force on the tip. (b) The sharp tip vibrates in a sinusoidal trajectory (dashed orange curve). If the ligand is bound to a receptor, the flexible spacer stretches upon retraction of the tip until the ligand unbinds (solid orange curve). The pulling forces drop to zero upon unbinding. The force measured before unbinding represents the strength of the receptor–ligand interaction. This entire process takes∼100 μs and the molecules are bound for a small fraction of this period. SMFS on the microsecond timescale We adapted the torsional harmonic cantilever concept for SMFS on the microsecond timescale using the scheme illustrated in Figure 1 . First, we attach the ligand to the tip of the T-shaped cantilever via a short flexible polymer strand and immobilize its binding partner on a substrate ( Fig. 1a ). Originally used for antibody recognition images, attaching the ligand to the tip of the AFM via a short flexible spacer has several benefits enabling high-speed SMFS [19] . It enhances binding probability by providing conformational flexibility for the ligand to reach the receptor and orient itself for binding. The flexible linker also provides a temporal delay between the tip–substrate interaction and the unbinding event [5] , [20] , which encodes the unbinding information onto the tip-sample force waveform. This information can be recovered by a computer that monitors the twisting motion of the T-shaped cantilever. Figure 1: Schematic of SMFS on the microsecond timescale. ( a ) The ligand is attached to a specially designed T-shaped AFM cantilever via a flexible polymer spacer. Tip-sample interactions twist the vibrating cantilever. The vertical deflection signal gives the tip position, and the twist angle gives the instantaneous force on the tip. ( b ) The sharp tip vibrates in a sinusoidal trajectory (dashed orange curve). If the ligand is bound to a receptor, the flexible spacer stretches upon retraction of the tip until the ligand unbinds (solid orange curve). The pulling forces drop to zero upon unbinding. The force measured before unbinding represents the strength of the receptor–ligand interaction. This entire process takes ∼ 100 μs and the molecules are bound for a small fraction of this period. Full size image Different from the previous design of the torsional harmonic cantilever, the scheme described in Figure 1b requires an ability to monitor forces at every single oscillation cycle with sufficient signal-to-noise ratio. 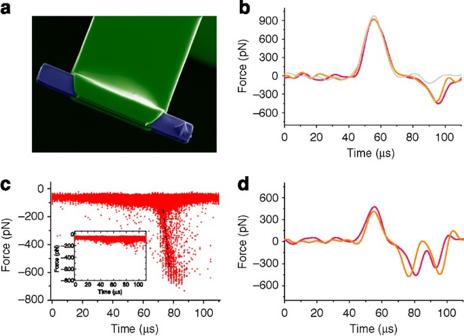Figure 2: Observation of microsecond timescale single-molecule interactions. (a) False colour electron microscopy image of a T-shaped cantilever designed for single-molecule experiments. Dimensions of the cantilever are given in the Methods section. (b) Examples of measured tip-sample force waveforms showing unbinding events of biotin and streptavidin using a 7-nm-long PEG spacer (orange and red curves). A force waveform recorded in the absence of streptavidin is given in grey. (c) A scatter plot formed by the lowest points of 105force waveforms. The times of unbinding events are determined mainly by the spacer length and vibration amplitude. These points are seen mostly between 70 and 90 μs. A linear fit to the data points in this region (dashed black line) estimates the force's rise with a rate of 102 pN μs−1. The inset incshows the scatter plot recorded after free biotin is added to the imaging buffer to block binding sites of streptavidin. The number of data points with forces below −200 pN reduced significantly. (d) Examples of force waveforms that exhibit multiple minima. We have designed the cantilever seen in Figure 2a that has force sensitivity sufficient to observe single-molecule interactions with adequate detail. With this cantilever, we have investigated the interaction of biotin with streptavidin adsorbed onto a mica substrate. A 7-nm-long polyethylene glycol (PEG) is used as the flexible linker. Two curves plotted in Figure 2b show the effect of unbinding on the force waveforms. The forces originating from the stretching of the spacer are observed between 80 and 95 μs. The lowest point in the force waveform approximately corresponds to the unbinding force; in the two cases seen in Figure 2b , these points are located near 95 μs. The rupture forces emerging from each pulling event are different because of the stochastic nature of unbinding. Figure 2: Observation of microsecond timescale single-molecule interactions. ( a ) False colour electron microscopy image of a T-shaped cantilever designed for single-molecule experiments. Dimensions of the cantilever are given in the Methods section. ( b ) Examples of measured tip-sample force waveforms showing unbinding events of biotin and streptavidin using a 7-nm-long PEG spacer (orange and red curves). A force waveform recorded in the absence of streptavidin is given in grey. ( c ) A scatter plot formed by the lowest points of 10 5 force waveforms. The times of unbinding events are determined mainly by the spacer length and vibration amplitude. These points are seen mostly between 70 and 90 μs. A linear fit to the data points in this region (dashed black line) estimates the force's rise with a rate of 102 pN μs −1 . The inset in c shows the scatter plot recorded after free biotin is added to the imaging buffer to block binding sites of streptavidin. The number of data points with forces below −200 pN reduced significantly. ( d ) Examples of force waveforms that exhibit multiple minima. Full size image Statistical distribution of the lowest forces obtained from repeatedly measured force waveforms is given in Figure 2c (examples of entire force waveforms and force-distance curves are given in Supplementary Movie 1 ). A large portion of measured forces does not exhibit binding and reflect measurement noise in the range of −40 to −100 pN. However, points with force values below −150 pN are mostly localized between 70 and 90 μs. These points also exhibit a trend in which larger pulling forces occur later. This trend is due to the stretching of the polymer spacer between the tip and the bound biotin–streptavidin complex that provides rapidly increasing forces as end to end distance approaches the contour length. As seen in the inset of Figure 2c , the number of data points in this region of the graph reduced significantly after adding free biotin to the imaging buffer to block binding sites of streptavidin molecules, providing evidence to the specificity of the measurements. A linear fit to data in the region below −150 pN estimates that the forces increase at a rate of 102 pN μs −1 . Considering that the pulling forces reach as much as 750 pN, we estimate the lifetime of the bound molecular complex to be around 4–8 μs. Discrimination of multiple unbinding events We note that forces as high as the ones measured here can be encountered in conventional SMFS experiments if multiple ligand–receptor interactions are formed and disrupted in one measurement cycle [7] . Multiple interactions are less likely to occur in the present measurements owing to the short period of oscillations. For biotin to bind streptavidin on the surface, the tip-sample distance has to be less than the length of the PEG spacer ( ∼ 7 nm). As the amplitude of the oscillations is 9 nm, binding has to occur in less than half the oscillation period ( ∼ 55 μs). Using the association constant determined from surface plasmon resonance measurements [21] (K a ≈5×10 6 M −1 s −1 ) and assuming an effective volume V eff ∼ 718 nm 3 for the tethered biotin (volume of a half sphere with 7-nm radius), we estimate the time that would lead to 50% binding probability to be ∼ 86 μs ( t 0.5 ≈ N A V eff / K a ) [19] . The binding probability is likely to be even lower than this estimate, because of the additional energy barrier imposed by the PEG spacer used in the experiment. Furthermore, owing to the high bandwidth (135 kHz) and effective spring constant (0.98 N m −1 ) of the torsional mode, multiple unbinding events within the same oscillation cycle can be potentially discriminated as multiple force minima. We have analysed a set of 2,300 force waveforms (all exhibiting a pulling force of more than 200 pN) and found only six such curves. Two of these curves are plotted in Figure 2d . Quantitative mapping of rapid single-molecule interactions The ability to perform SMFS at each cycle of the oscillating cantilever permits mapping of molecular interaction forces quantitatively across surfaces. 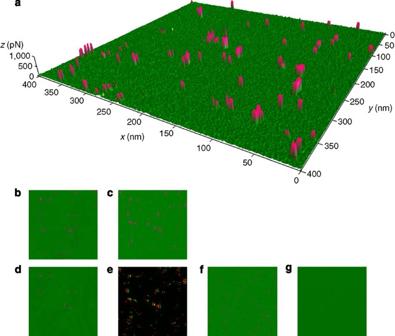Figure 3: Imaging rapid single-molecule interactions. (a) Spatially resolved pulling forces recorded across streptavidin molecules sparsely distributed on a mica substrate. Forces are coded into height (zaxis) and colour. Unbinding events appear as spikes because the corresponding forces are significantly larger than background. Topography, force map and phase image are given in (b–d), respectively. Scan size is 400 nm. Height values above 0.5 nm, phase values above 2° with respect to background and force values above 200 pN are given in pink. To compare the force maps recorded in trace and retrace directions, force spikes in each image are overlaid (e), with the green spots corresponding to trace and red spots corresponding to retrace. Although trace and retrace images are not identical, there is a strong correlation. The slight offset is due to the delay introduced during the online data analysis (trace images shift slightly right and retrace images shift slightly left). The phase image inddoes not show as many features as the force maps or the topography. After the addition of free biotin to the imaging buffer, topographical features remained (f), but force spikes disappeared (g). Scan size infandgis 4 μm. Figure 3a demonstrates one such image generated by mapping the maximum pulling forces across a 400-nm-wide region of the sample. We observe that the unbinding forces are well above the noise floor so that they appear as clear spikes. This is a direct consequence of the specificity of the information provided by SMFS. The spikes generated by the distinct interaction forces are locating the receptor molecules within ∼ 7 nm, because the ligand can bind to a receptor within that radius. A comparison of the force map to the simultaneously recorded topography image ( Fig. 3b,c ) shows that the locations of the force spikes correlate well with topographical features. A force map obtained with another tip-sample combination also exhibited this characteristic ( Supplementary Fig. S1 ). We note that, a number of force spikes do not have a corresponding topographical feature. These may represent unspecific interactions or detachment of streptavidin molecules from the surface. We have also recorded the conventional phase image, simultaneously ( Fig. 3d ). The phase image does not show as many features as the force map or topography. Phase signal is sensitive to mechanical properties of the surface. Therefore, the features in the phase signal are likely originating from aggregated streptavidin, which can create larger mechanical contrast. Note that the topographical features corresponding to those locations are wider than other topographical features. We also observed that the locations of the force spikes recorded in trace and retrace directions correlate strongly ( Fig. 3e ). In addition, these force spikes disappeared after introducing biotin to the imaging buffer to block binding sites ( Fig. 3f,g ). These observations show that microsecond timescale single-molecule interactions can be quantitatively measured and spatially mapped with high resolution. Figure 3: Imaging rapid single-molecule interactions. ( a ) Spatially resolved pulling forces recorded across streptavidin molecules sparsely distributed on a mica substrate. Forces are coded into height ( z axis) and colour. Unbinding events appear as spikes because the corresponding forces are significantly larger than background. Topography, force map and phase image are given in ( b–d ), respectively. Scan size is 400 nm. Height values above 0.5 nm, phase values above 2° with respect to background and force values above 200 pN are given in pink. To compare the force maps recorded in trace and retrace directions, force spikes in each image are overlaid ( e ), with the green spots corresponding to trace and red spots corresponding to retrace. Although trace and retrace images are not identical, there is a strong correlation. The slight offset is due to the delay introduced during the online data analysis (trace images shift slightly right and retrace images shift slightly left). The phase image in d does not show as many features as the force maps or the topography. After the addition of free biotin to the imaging buffer, topographical features remained ( f ), but force spikes disappeared ( g ). Scan size in f and g is 4 μm. 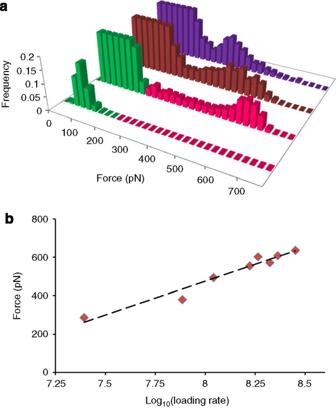Figure 4: Loading rate dependency at short timescales. (a) Histograms generated from pulling forces. Forces recorded inFigure 3aare plotted at two different scales to show the peak corresponding to noise (first row, frequency values are divided by 250 to fit into the same plot area) and the peak corresponding to the most likely rupture force of biotin–streptavidin complex at 625 pN (second row). The data show unbinding forces as high as 750 pN. Additional histograms generated at gradually reduced loading rates are given in brown and purple. The loading rate is reduced by lowering the oscillation amplitude. (b) Most likely rupture forces measured at various loading rates. Linear fit to the data points is given with the black dashed curve. Loading rates are in units of pN sec−1. The slope of the linear fit corresponds to a barrier position ofxβ≅0.27 Å. Full size image Statistics of rupture forces Histograms generated from the pulling forces recorded while the cantilever scans the surface are given in Figure 4a . Each histogram exhibits two peaks. The first peak at the lower force level corresponds to the background determined by unspecific interactions and measurement noise (first row in Fig. 4a ). The second peak is seen only after adjusting the scale of the frequency axis (second row in Fig. 4a ). This is because most oscillation cycles do not result in biotin–streptavidin binding. Note that the histograms in the first and second rows correspond to the measurements in Figure 3a . According these measurements, the majority of rupture forces are around 625 pN. Forces as much as 750 pN are measured as well. These values are much higher than the rupture forces previously reported for this molecular complex [7] , [15] , [22] , [23] , which is a consequence of the significantly higher loading rate achieved. Figure 4: Loading rate dependency at short timescales. ( a ) Histograms generated from pulling forces. Forces recorded in Figure 3a are plotted at two different scales to show the peak corresponding to noise (first row, frequency values are divided by 250 to fit into the same plot area) and the peak corresponding to the most likely rupture force of biotin–streptavidin complex at 625 pN (second row). The data show unbinding forces as high as 750 pN. Additional histograms generated at gradually reduced loading rates are given in brown and purple. The loading rate is reduced by lowering the oscillation amplitude. ( b ) Most likely rupture forces measured at various loading rates. Linear fit to the data points is given with the black dashed curve. Loading rates are in units of pN sec −1 . The slope of the linear fit corresponds to a barrier position of x β ≅ 0.27 Å. Full size image Varying the loading rate We have varied the loading rate by reducing the vibration amplitude at a constant oscillation frequency and observed the resulting changes in the values of most likely rupture forces (third and fourth rows in Fig. 4a ). The histograms in the second, third and fourth rows are recorded at 9, 6 and 4.5 nm, respectively. We estimated the loading rates by linearly fitting the force versus time plots as in Figure 2c . Figure 4b shows the most likely rupture forces plotted against the loading rate. The loading rate dependency of most likely rupture forces contains information about the energy landscape of receptor–ligand interactions. When measured over a wide dynamic range and plotted on a logarithmic scale, different energy barriers can be resolved from the changes in the slope [15] , [24] , [25] . The position of the barrier x β is related to the slope f β by f β =k B T / x β (here k B is Boltzmann constant and T is temperature) [24] , [26] . According to this formulation, the slope of the forces measured here corresponds to a barrier position x β ≅ 0.27 Å. The barrier position derived from the loading-rate-dependant measurements are considerably smaller than previous estimates of the innermost barrier position [15] of 1.2 Å, suggesting the possibility of an additional barrier. This is also supported by the results of Zhou et al . [27] , combined MD and continuum mechanics simulations of which identified barriers at 0.3, 1.0 and 2.6 Å. According to their simulations, the innermost barrier is maintained by two hydrogen bonds to biotin by Thr90 and Asn49 of streptavidin. Note that steered MD simulations of other protein materials also revealed barrier positions comparable to the one measured here [16] . Recent theoretical and experimental works showed that the stiffness of the force transducer can influence the measured rupture forces [28] , [29] . Using analytical models generalized to include stiff transducers, Maitra and Arya [29] have found that the comparison of rupture force spectra obtained with different devices is permissible if spring constants K and barrier positions x β satisfy the relationship Kx 2 β /(2 k B T ) ≪ 1. In the present experiment, forces are measured by the torsional deflections, of which the effective spring constant at the position of the offset tip is ∼ 0.98 N m −1 . Using x β ≅ 0.27 Å, we obtain Kx 2 β /(2 k B T ) ≅ 0.08. Note that the effective spring constant can be even lower because of the presence of the linker attaching biotin to the tip. Therefore, we argue that the measured x β corresponds to an additional barrier in the energy landscape of biotin–streptavidin. In addition to the evidence provided for an additional energy barrier, the data also provide experimental evidence that the forces can be as high as that predicted by MD simulations [14] . Those calculations identified several unbinding paths for avidin–biotin complex, with rupture forces between 650 and 800 pN. The MD simulations were carried out on a timescale on the order of 1 ns; however, recent MD simulations now reach hundreds of nanoseconds [16] , [30] . As a result, the timescales of experiments and simulations are now within about an order of magnitude. This gap can be bridged with the use of small AFM cantilevers, as Ando et al . [31] demonstrated a small cantilever AFM system that can detect torsional vibrations while the cantilever was driven at 1 MHz. The rapid nanomechanical interface presented here can have various applications beyond probing the energy landscapes of receptor–ligand interactions. For example, cut-and-paste-based molecular assembly schemes rely on selective formation and rupture of a series of chemical bonds between an ink molecule with the carrier tip and the surfaces of depot or target areas [10] . Theoretical calculations have shown that when chemical bonds in series are subject to external force, loading rate can selectively determine which bond will break first [32] . This rate-dependent behaviour would allow picking up molecular inks at one loading rate and delivering them at another loading rate using a universal chemistry at the depot and target surfaces, which would also permit reversible rearrangements of assembled structures. This can potentially be realized experimentally by switching between conventional SMFS and the high-speed approach presented here. Variability in bond rupture mechanisms at different loading rates or timescales has biological implications as well. MD simulations of protein building blocks demonstrated variations in failure mechanisms in response to loading rates [16] . Experiments with the rapid nanomechanical interface presented here can provide new insights to deformation and failure mechanisms of protein-based materials like collagen and silk, strengths of which are critical for their biological functions [33] . Experiments also afford greater control of the environment so that effects of solvent pH and ionic strength can be investigated in depth. Torsional harmonic cantilevers T-shaped cantilevers are fabricated by using conventional manufacturing protocols (Applied Nanostructures) with custom geometry. The body of the cantilever is made of silicon nitride and the wider region at the free end including the tip is made of silicon. The probes are 130-μm long and 35-μm wide. The width at the free end is 55 μm. The tip offset distance is 22 μm (measured by electron microscopy). The thickness of the silicon nitride is 600 nm. It has 30-nm-thick gold coating. The thickness of the silicon part is ∼ 1 μm. The resonance frequencies of these cantilevers in solution are around 9.5 kHz, determined from the thermal noise spectrum. Their torsional resonances and quality factors are ∼ 115 kHz and 3.5, respectively. The force sensitivity of the torsional mode is calibrated against the thermal noise and found to be 8.0 nN V −1 . This corresponds to an effective spring constant of 0.98 N m −1 (defined by ratio of the tip displacement in the torsional mode to the force acting on the tip). Experimental setup A commercial AFM system (Multimode series with a Nanoscope 5 controller, and a signal breakout box) has been used. Measurements and imaging are done in fluid tapping mode. The T-shaped cantilever is driven at 9 kHz. Vibration amplitude was set to 4.5, 6 or 9 nm. Cantilever vibration signals are collected with a personal computer equipped with two processors (3.2 GHz, 2 GB shared memory) and a data acquisition card (NI-DAQ S-series 6115). Calculations of tip-sample force waveforms from the torsional vibration signals are carried out in Labview (National Instruments). We followed the same procedures reported previously [17] to invert the transfer function of the torsional mode and eliminate cross talk from large vertical deflection signals; however, every oscillation cycle is analysed individually. This approach is based on a framework used by Stark et al . [34] for the analysis of higher harmonic vibrations. In a previous work [35] , we have tested tip-sample force waveforms generated from the torsional vibrations by comparing the measured forces with the previously developed theories [36] , [37] of cantilevers vibrating in the tapping mode. See also Solares and Hoelscher [38] for numerical analysis of the measurements based on torsional harmonic cantilever. In the calculations made here, torsional vibration signals up to 135 kHz are included. At a typical scan speed of 1 Hz, approximately nine oscillation cycles are analysed per pixel of the AFM image. The lowest force value measured in those nine cycles is recorded at that pixel to generate unbinding force maps as in Figure 3a . Tip modification T-shaped cantilevers are cleaned in an O 2 plasma for 5 min and then transferred to a piranha solution (sulphuric acid/H 2 O 2 , 8:2) for 30 min. After extensive rinsing with nanopure H 2 O, the tips are transferred into a fresh ethanol solution, which contains 5% APTES (3-aminopropy-triethoxysilane; Sigma Aldrich), 5% de-ionized water and 90% absolute ethanol, for 30 minutes at room temperature. The amino-functionalized AFM tips are rinsed with de-ionized water five times and pure ethanol five times, followed by drying with a gentle stream of nitrogen. Next, carboxyl-group polyethylene oxide PEG polymers with biotin end groups (Biotin PEG propionic acid, C 37 H 69 N 3 O 16 S, Polypure AS) were covalently linked to the silanized AFM tip surfaces using Polylink protein coupling kit (Bangs Laboratories). The Biotin-PEG-COOH was diluted in coupling buffer (50 mM MES, pH 5.2, 0.05% Proclin300). The EDAC (carbodiimide) solution was prepared by dissolving EDAC in coupling buffer. AFM tips were incubated in the mixture solution of Biotin-PEG-COOH and EDAC for 45 min at room temperature. Right after incubation, Biotin-functionalized AFM tips were rinsed with washing buffer (10 mM Tris, pH 8.0 bovine serum albumin, 0.05% Proclin300) for three times. Sample preparation A stock solution of streptavidin (Sigma Aldrich) in 1 mg ml −1 PBS was diluted with 100 mM NaCl to a final streptavidin concentration of 0.8 μg ml −1 . Fresh-cleaved mica was incubated with streptavidin solution for 20 min and subsequently rinsed with PBS buffer solution for two times. The mica sheet was mounted in a fluid cell for AFM experiments. Measurements are carried out in PBS. Testing the specificity of interaction forces Specificity of the measured rupture forces is tested by blocking the binding sites of immobilized streptavidin molecules with free biotin introduced into the imaging buffer. The results are given in Figure 3 . How to cite this article: Dong, M. & Sahin, O. A nanomechanical interface to rapid single-molecule interactions. Nat. Commun. 2:247 doi: 10.1038/ncomms1246 (2011).